A source of antihydrogen for in-flight hyperfine spectroscopy Antihydrogen, a positron bound to an antiproton, is the simplest antiatom. Its counterpart—hydrogen—is one of the most precisely investigated and best understood systems in physics research. High-resolution comparisons of both systems provide sensitive tests of CPT symmetry, which is the most fundamental symmetry in the Standard Model of elementary particle physics. Any measured difference would point to CPT violation and thus to new physics. Here we report the development of an antihydrogen source using a cusp trap for in-flight spectroscopy. A total of 80 antihydrogen atoms are unambiguously detected 2.7 m downstream of the production region, where perturbing residual magnetic fields are small. This is a major step towards precision spectroscopy of the ground-state hyperfine splitting of antihydrogen using Rabi-like beam spectroscopy. Within the Standard Model of particle physics, CPT symmetry is conserved and the spectroscopic properties of antihydrogen ( ) and its counterpart hydrogen are predicted to be identical. Thus, precise comparisons between hydrogen and its antimatter counterpart provide sensitive tests of CPT invariance. Historically, the high-precision spectroscopy of hydrogen inspired the development of numerous elegant experimental methods. This culminated in frequency-comb-locked optical two-photon spectroscopy of the 1 S –2 S transition, where the remarkable precision of 4.2 × 10 −15 was achieved [1] , corresponding to an absolute frequency resolution of 10 Hz. Other experimental efforts focused on precision spectroscopy of the ground-state hyperfine splitting (GS-HFS) by using a hydrogen maser. Here the GS-HFS transition frequency v HFS of ~1.4 GHz was measured with an absolute precision of 1 mHz (ref. 2 ), which corresponds to a relative precision of 7.0 × 10 −13 . The goal of our experiment is the precise measurement of the antihydrogen GS-HFS [3] . In the framework of the so-called Standard Model Extension (SME) [4] , which is an extension of the Standard Model allowing Lorentz and CPT violations, GS-HFS spectroscopy of hydrogen and antihydrogen provides one of the most sensitive tests of CPT symmetry. In addition, the SME predicts that while GS-HFS is directly sensitive to the CPT violating terms, in the case of the 1 S –2 S transition frequency it is only a second-order effect. In contrast to the table-top matter experiments, antihydrogen spectroscopy requires complex apparatuses for the production of the elusive antimatter atoms. In addition, antihydrogen atoms cannot be confined in a container made out of matter because they immediately annihilate. To overcome this difficulty, the ALPHA and the ATRAP collaborations at the Antiproton Decelerator (AD) of CERN plan spectroscopy of confined in magnetic traps with an effective potential depth of only ~40 μeV. Recently both collaborations reported the trapping of ground-state (refs 5 , 6 , 7 ). Moreover, the ALPHA collaboration observed hyperfine transitions induced in trapped antihydrogen atoms [8] . However, trapping of requires strong magnetic field gradients, which broaden the transition line-widths and reduce experimental precision. Thus, we adopt an alternative strategy: the Rabi-like spectroscopy of antihydrogen GS-HFS [9] , which is based on polarized antiatomic beams. This scheme uses a so-called cusp trap [10] , [11] , which is a combination of the magnetic field of a unique superconducting anti-Helmholtz coil assembly and multiple ring electrodes (MRE) for the electrostatic manipulation of trapped non-neutral plasmas. The magnetic field gradient produced by the cusp magnetic field exerts a force on the antihydrogen atoms. Low-field-seeking states are preferentially guided along the cusp trap axis, whereas high-field seekers are de-focused [10] , resulting in a spin-polarized beam. The atoms are then passed through a microwave cavity, focused by a spin-selector (a sextupole magnet) and finally detected by an antihydrogen detector. When the microwave frequency is equal to the hyperfine transition frequency, the low-field-seeking states are converted to high-field-seeking states and de-focused by the sextupole magnet. In contrast to the spectroscopic techniques based on trapped antihydrogen, antiatoms of several meV energy can be guided to a region with a weak magnetic field. This allows in-flight precision spectroscopy at the level of 10 −7 or better [12] . While the 1 S –2 S transition is primarily an electric phenomenon, the hyperfine structure is predominantly of magnetic origin. It is mainly caused by the interaction of the magnetic moments of the positron and the antiproton . The ground state splits into two substates: for parallel magnetic moments ( F =0, singlet state) the effective two-body interaction potential is attractive, while repulsive in the other case ( F =1, triplet state). The zero-field F =0→ F =1 transition frequency v HFS is first-order proportional to the direct product of and . The Zemach and nuclear polarizability corrections lead to a deviation from the first-order calculation at a level of ~40 p.p.m. [13] Combined with independent measurements of the proton and antiproton magnetic moments [14] , [15] , the precise determination of the GS-HFS provides constraints on CPT symmetry of the electric and magnetic form factors of the two particles. This constitutes an additional CPT symmetry test of the internal structure of protons and antiprotons. This Article describes the development of an antihydrogen source using a cusp trap for Rabi-like beam spectroscopy. A significant fraction of antihydrogen atoms in quantum states below n =29 are detected at 2.7 m downstream of the production region, where perturbing residual magnetic fields are small. The antihydrogen number per hour is estimated to be ~25. This is an important milestone towards the planned precision spectroscopy of the GS-HFS of antihydrogen. Experimental set-up To achieve our physics goal, we have developed the experimental apparatus shown in Fig. 1 . It consists of an ultra-slow antiproton beam source (MUSASHI) [16] , a positron accumulator [17] , ultra-low energy beam transport lines and the cusp trap, which is a superposition of the strong magnetic field gradient provided by the superconducting anti-Helmholtz coil and an electrostatic potential [10] . For the preparation of antiproton and positron plasmas Penning–Malmberg type traps are used. They comprise a homogeneous strong axial magnetic field and an electrostatic potential. In all cases MRE [18] are introduced into the respective magnets for the electrostatic manipulation of the trapped plasmas. Two scintillator modules are placed on each side of the cusp magnet, which are utilized to track pions produced by antiproton annihilation. This pion-tracking detector provides information about the antiproton annihilation position distribution. Downstream of the cusp trap a hyperfine spectrometer line is placed. It consists of a microwave cavity to induce spin flips, a superconducting sextupole magnet for spin-state analysis and an antihydrogen detector [19] . In the experiments described in this article, the microwave cavity is not used and the detector is placed 2.7 m downstream of the production region. 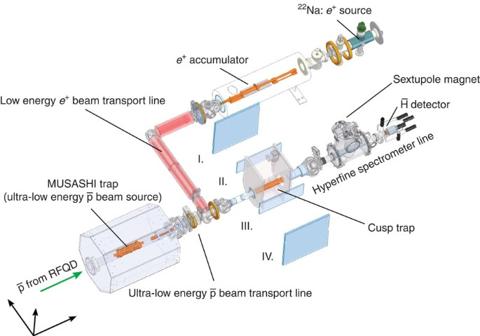Figure 1: Schematic view of our experimental apparatus. Arrows represent 1 m in each direction. Antiprotons delivered from the AD via the RFQD are trapped, electron-cooled and radially compressed in the MUSASHI. Moderated positrons from a22Na source are prepared and cooled in the positron accumulator and then are transported to the cusp trap. The cusp trap consists of an MRE and superconducting anti-Helmholtz coils. After positrons are accumulated near the maximum magnetic field region, antiprotons are injected from the MUSASHI and mixed with positrons synthesizing antihydrogen atoms. Antihydrogen atoms in low-field-seeking states are focused downstream of the cusp trap due to the strong magnetic field gradient, while those high-field-seeking states are de-focused. Thus, a polarized antihydrogen beam is produced. On both sides of the cusp trap, scintillator modules labelled as I–IV are mounted, which are used to track charged pions produced by annihilation reactions. Downstream of the cusp trap a spectrometer line is placed, which involves a sextupole magnet and an antihydrogen detector. Figure 1: Schematic view of our experimental apparatus. Arrows represent 1 m in each direction. Antiprotons delivered from the AD via the RFQD are trapped, electron-cooled and radially compressed in the MUSASHI. Moderated positrons from a 22 Na source are prepared and cooled in the positron accumulator and then are transported to the cusp trap. The cusp trap consists of an MRE and superconducting anti-Helmholtz coils. After positrons are accumulated near the maximum magnetic field region, antiprotons are injected from the MUSASHI and mixed with positrons synthesizing antihydrogen atoms. Antihydrogen atoms in low-field-seeking states are focused downstream of the cusp trap due to the strong magnetic field gradient, while those high-field-seeking states are de-focused. Thus, a polarized antihydrogen beam is produced. On both sides of the cusp trap, scintillator modules labelled as I–IV are mounted, which are used to track charged pions produced by annihilation reactions. Downstream of the cusp trap a spectrometer line is placed, which involves a sextupole magnet and an antihydrogen detector. Full size image Antiprotons at 5.3 MeV from the AD pass a radio-frequency quadrupole decelerator (RFQD) that reduces their energy to 115 keV. Subsequently, the particles transmit through thin degrader foils (two 90 μg cm −2 biaxially oriented polyethylene terephtalate foils) [20] and are trapped in the MUSASHI antiproton trap. The unique scheme of sequential combination of the RFQD and the MUSASHI trap enables us to use 5–50 times more antiprotons (over 10 6 in number) per AD cycle than other antihydrogen experiments [16] . In the MUSASHI trap the antiprotons are electron-cooled and radially compressed by a rotating electric field [21] . This preparation procedure enables the efficient transfer of an ultra-low energy antiproton beam to the cusp trap [16] . Positrons are provided from a 22 Na source with an activity of 0.6 GBq. The particles are moderated by Ne ice grown on a small cone in front of the source [22] , [23] . By interaction with a N 2 /CF 4 gas mixture the positrons are trapped and further thermalized in the MRE of the positron accumulator. Subsequently, the accumulated particles are transferred to the cusp trap. By repeating this sequence, typically 3 × 10 7 positrons are loaded into the cusp magnet in ~10 min. Antihydrogen production in the cusp trap For the production of antihydrogen atoms a nested well configuration is employed [24] , [25] , [26] , as shown in Fig. 2a , located in the local maximum of the cusp magnetic field. Simulations predict that when the mixing of positrons and antiprotons is performed at this position, the cusp magnetic field enhances the polarization of atoms, which flow out towards the downstream direction and pass the magnetic field minimum. About 3 × 10 5 antiprotons from the MUSASHI trap are injected into the positron plasma stored in the nested well. The kinetic energy of the antiproton beam is adjusted to be slightly above the potential energy of the plasma ( Fig. 2a ) in order to avoid significant heating induced by the antiproton injection. In contrast to the charged particles confined in the nested well, electrically neutral antihydrogen atoms escape from this potential configuration. 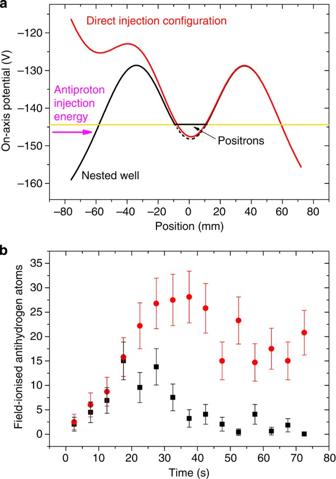Figure 2: Antihydrogen synthesis. (a) Illustration of the direct injection scheme, which is used to produce antihydrogen atoms. A positron plasma is confined and compressed at the centre of the nested well (black solid line). The potential is opened (red solid line) when antiprotons with low energy spread are injected into the positron plasma. The antiproton kinetic energy is adjusted to slightly higher than the potential energy of the positron plasma (yellow solid line), which ensures efficient mixing of antiprotons and positrons. To prolong the interaction time during mixing, an rf drive (not shown in the figure) is applied, which drives the axial oscillation of the antiprotons. (b) The number of antihydrogen atoms field-ionized downstream of the nested trap as a function of time. The filled black squares are from an experiment when direct injection was applied. The filled red circles represent results obtained from the rf-assisted direct injection scheme. Error bars show s.d. of the mean. By applying the rf drive the yield of field-ionized antihydrogen atoms was increased by a factor of 3.5. Figure 2: Antihydrogen synthesis. ( a ) Illustration of the direct injection scheme, which is used to produce antihydrogen atoms. A positron plasma is confined and compressed at the centre of the nested well (black solid line). The potential is opened (red solid line) when antiprotons with low energy spread are injected into the positron plasma. The antiproton kinetic energy is adjusted to slightly higher than the potential energy of the positron plasma (yellow solid line), which ensures efficient mixing of antiprotons and positrons. To prolong the interaction time during mixing, an rf drive (not shown in the figure) is applied, which drives the axial oscillation of the antiprotons. ( b ) The number of antihydrogen atoms field-ionized downstream of the nested trap as a function of time. The filled black squares are from an experiment when direct injection was applied. The filled red circles represent results obtained from the rf-assisted direct injection scheme. Error bars show s.d. of the mean. By applying the rf drive the yield of field-ionized antihydrogen atoms was increased by a factor of 3.5. Full size image To monitor antihydrogen synthesis, we prepare a field ionization well 20 cm downstream of the mixing region [11] . An antihydrogen atom in a Rydberg state with principal quantum number n is field-ionized if n ⩾ (3.2/ ε ) 1/4 × 10 2 is satisfied [27] , where ε (V cm −1 ) is the electric field strength. The average field strength is 139 V cm −1 (93 V cm −1 on axis), which can field-ionize antihydrogen atoms with n ≳ 39. Here we define the average electric field strength, which is the mean value of the field averaged over the entire trap radius. Resulting antiprotons are trapped in the field-ionization well [11] , [26] . When this well is opened, the particles escape from the trap, annihilate and are counted by the pion-tracking detector. In such a direct injection scheme typically 75 field-ionization counts are obtained in a time interval of 80 s. To investigate the time evolution of antihydrogen formation, during the mixing process the field ionization well is opened and closed periodically. Results of that measurement are shown in Fig. 2b (filled squares). A maximum is reached after ~20 s, followed by a slow decrease explained by the axial separation of antiprotons and positrons. This separation is due to two possible processes: one process is the energy loss of the antiprotons by interaction with electrons formed in annihilation with the background gas; the other is the reduction of the antiproton’s axial energy due to collisional relaxation. When the axial energy of the antiprotons drops below the positron potential energy, the synthesis is stopped. This axial separation model is based on information obtained from our position-sensitive pion-tracking detector [11] . To counteract the axial separation and to prolong the antihydrogen production period, an rf-assisted direct injection scheme was developed. During the mixing process an rf drive at 420 kHz is applied to one of the ring electrodes of the MRE, which excites the axial oscillation of the trapped antiprotons [28] . The filled red circles in Fig. 2b represent a typical result obtained from such an experiment. More than 260 antiprotons are counted in the time-window of 80 s, which is a factor of 3.5 more than without rf. Detection in a magnetic field-free environment The antihydrogen detector placed at the end of the spectrometer line is made out of a bismuth germanium oxide (Bi 4 Ge 3 O 12 , BGO) single-crystal. This scintillating material was selected because of its high density (7.13 g cm −3 ), high photon yield (8–10 per keV energy deposit) and ultra-high vacuum compatibility. The BGO crystal has a diameter of 10 cm and a thickness of 5 mm. It is placed inside a vacuum chamber with its centre on the beam axis. Outside the chamber, five plastic scintillator plates (thickness 10 mm, total solid angle coverage 49% of 4π) are installed to detect annihilation pions. Each scintillator is read-out by a photomultiplier tube. The BGO signal is recorded by a waveform digitizer while the timing of the plastic scintillator signal is read-out by time-to-digital converters. The signal of the BGO scintillator was energy calibrated by comparing measured cosmic rays with simulations using GEANT4 (ref. 29 ) and the CRY package [30] . Antiproton annihilations originating from antihydrogen atoms hitting the crystal surface yield on average three charged pions with a mean momentum of ~300 MeV c −1 (ref. 31 ), which are detected by the plastic scintillators. In order to reduce background events from antiprotons annihilating upstream or from cosmic rays, a coincidence between the BGO and the plastic scintillators is required. Owing to the high multiplicity of the annihilation products, coincidence with at least two plastic scintillators can be used. According to our simulations this coincidence condition reduces the background event rate by three orders of magnitude while the signal count rate is only reduced by about a factor of 2. Using even higher multiplicities leads to an additional decrease of the signal by at least a factor of 3. Thus double coincidence events are used in the following analysis. To investigate the principal quantum number of the antihydrogen atoms that reach the detector, voltages of either −400 or −2,000 V are applied to a set of field-ionization electrodes located in front of the BGO scintillator, which corresponds to average electric fields of 94 V cm −1 ( n ≳ 43) and 452 V cm −1 ( n ≳ 29), respectively (hereafter called scheme 1 and scheme 2). In other words, the antihydrogen atoms with n ≲ 43 (scheme 1) or n ≲ 29 (scheme 2) reach the BGO scintillator, while the antiprotons originating from field-ionized antihydrogen are repelled by the electric field. The unshaded histogram bordered by the solid line in Fig. 3a shows the distribution of energy deposited in the BGO scintillator for double coincidence events up to 200 MeV for scheme 1. According to simulations, 200 MeV is the maximum energy deposited on the BGO scintillator when an antiproton annihilates on its surface. The shaded histogram shows results where antiprotons are trapped and cooled with electrons instead of positrons (referred to as a background run hereafter). The obtained energy spectrum represents events originating from cosmic rays and secondary particles, especially charged pions, which are produced by annihilation of antiprotons trapped in the nested well. The annihilation rate during the background run is expected to be comparable to the background annihilation rate of schemes 1 and 2. As in the low-energy region the annihilation cross section S is proportional to 1/ ν (Langevin cross section), the annihilation rate, which is proportional to νS , does not depend on the antiproton energy, where ν is the relative velocity between the antiproton and a residual gas atom [32] . A GEANT4 simulation predicts that events due to antihydrogen annihilation along the vacuum tube upstream of the BGO scintillator are negligibly small. 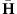Figure 3: Energy deposition byatoms and estimated number ofatoms. (a) Distributions of energy deposition in the BGO scintillator for the double coincidence condition (see the text). The distributions are normalized to one mixing cycle of 150 s. The unshaded histogram bordered by the thick blue line is obtained from scheme 1. The total data accumulation time was 4,950 s. The shaded histogram represents data obtained from the background runs, in a total time of 1,550 s. A clear difference is seen at energies higher than 40 MeV, indicating the observation of antihydrogen atoms. (b) The number of integrated events as a function of threshold energy,Eth, after subtraction of the background events. Filled squares are for scheme 1, filled triangles for scheme 2. Errors are propagated from the s.d. of the observed event numbers. (c) The estimated number of antihydrogen atoms that reached the BGO scintillator. The numbers are evaluated by calibrating the counts shown inbwith the detection probability as a function ofEthpredicted by GEANT4 simulation. Figure 3a shows that the number of events with energy deposition above 40 MeV are significantly larger than those of the background run, that is, the threshold energy E th =40 MeV can be chosen to identify antihydrogen atoms annihilating on the BGO scintillator. The total accumulation times for the schemes 1 and 2, and a background run were 4,950, 2,100 and 1,550 s, respectively. Figure 3: Energy deposition by atoms and estimated number of atoms. ( a ) Distributions of energy deposition in the BGO scintillator for the double coincidence condition (see the text). The distributions are normalized to one mixing cycle of 150 s. The unshaded histogram bordered by the thick blue line is obtained from scheme 1. The total data accumulation time was 4,950 s. The shaded histogram represents data obtained from the background runs, in a total time of 1,550 s. A clear difference is seen at energies higher than 40 MeV, indicating the observation of antihydrogen atoms. ( b ) The number of integrated events as a function of threshold energy, E th , after subtraction of the background events. Filled squares are for scheme 1, filled triangles for scheme 2. Errors are propagated from the s.d. of the observed event numbers. ( c ) The estimated number of antihydrogen atoms that reached the BGO scintillator. The numbers are evaluated by calibrating the counts shown in b with the detection probability as a function of E th predicted by GEANT4 simulation. Full size image To evaluate the statistical significance of these results, the measured energy deposition spectra are integrated from E th to 200 MeV. The filled squares and filled triangles in Fig. 3b show such integrated events after subtraction of background counts for both schemes, normalized to the data accumulation time of 150 s. Taking into account the detection probability as a function of E th predicted by GEANT4, the absolute number of antihydrogen atoms arriving at the BGO scintillator was evaluated, which is shown in Fig. 3c . Irrespective of the threshold energy, for both schemes the numbers are almost constant. We obtain around 6 and 4 for schemes 1 and 2, respectively. This demonstrates that the characteristics of the detector system are well understood and under full control. In Table 1 the results of the analysis are summarized. It shows the total measurement time, the total number of double coincidence events N t , the total number of double coincidence events with deposition energy higher than 40 MeV in the BGO scintillator N >40 and the statistical significance of N >40 . In the case of scheme 1, we detected 99 candidate events in 4,950 s, while 6 is the observed number of background events in 1,550 s. The statistical significance of our data was evaluated using the following two methods. The profile likelihood significance incorporating Poisson fluctuations in the data [33] is 5.0 σ . The Z -value (significance in one-sided Gaussian standard deviations) for the ratio of Poisson means [34] is 4.8 σ . These statistical significances unambiguously prove the observation of antihydrogen atoms with n ≲ 43 at a distance of 2.7 m downstream of the antihydrogen production region. Furthermore, in the case of scheme 2, in total, 29 events in 2,100 s are detected, while 6 background events in 1,550 s are observed as well. The statistical significance for scheme 2 becomes 3.0 σ ( Z -value). This clearly indicates that a significant fraction of the observed antihydrogen atoms are in quantum states n ≲ 29. The expected antihydrogen number per mixing cycle for schemes 1 and 2 is around 6 and 4, respectively. Considering the fact that the total time per mixing cycle is ~15 min, the intensity values for schemes 1 and 2 are estimated to be ~25 and 16 per hour, respectively. It is noted that the observed principal quantum numbers are upper limits, constrained by the utilized field-ionization technique. Further quantum state analysis as well as the investigation of mechanisms for efficient de-excitation of Rydberg antihydrogen will be the scope of future research activities. The latter constitutes a significant, widely recognized challenge in the field of antihydrogen research [35] , [36] , [37] . Table 1 Summary of antihydrogen events detected by the antihydrogen detector. Full size table In conclusion, we have developed a source for the in-flight GS-HFS spectroscopy of antihydrogen. We detected a significant fraction of antihydrogen atoms in quantum states below n =29 at 2.7 m downstream of the production region. This opens the way towards a variety of other attractive physics experiments such as optical spectroscopy [38] , [39] and studies of the weak equivalence principle [40] , [41] . How to cite this article: Kuroda, N. et al . A source of antihydrogen for in-flight hyperfine spectroscopy. Nat. Commun. 5:3089 doi: 10.1038/ncomms4089 (2014).